Observing chaos for quantum-dot microlasers with external feedback Chaos presents a striking and fascinating phenomenon of nonlinear systems. A common aspect of such systems is the presence of feedback that couples the output signal partially back to the input. Feedback coupling can be well controlled in optoelectronic devices such as conventional semiconductor lasers that provide bench-top platforms for the study of chaotic behaviour and high bit rate random number generation. Here we experimentally demonstrate that chaos can be observed for quantum-dot microlasers operating close to the quantum limit at nW output powers. Applying self-feedback to a quantum-dot microlaser results in a dramatic change in the photon statistics wherein strong, super-thermal photon bunching is indicative of random-intensity fluctuations associated with the spiked emission of light. Our experiments reveal that gain competition of few quantum dots in the active layer enhances the influence of self-feedback and will open up new avenues for the study of chaos in quantum systems. Advances in semiconductor nanotechnology have triggered considerable research and development of photonic devices in the quantum limit. Of particular interest are structures based on quantum dots (QDs) which can act as two level quantum emitters in single photon sources [1] and sources of entangled photons [2] for future quantum communication networks [3] . In state-of-the art microlasers, cavity quantum electrodynamics ensures that a large fraction, β , of the spontaneous emission is coupled into the lasing mode. This makes it possible to design microlasers with ultra-low thresholds and a few QDs or even a single QD as gain medium [4] , [5] , [6] , [7] , [8] , [9] . As a result, the laser operation can be disturbed by the emission of single photons, which is reflected in dynamical antibunching in the photon statistics of the emitted light [10] . The sensitivity of quantum dot-microlasers on the particular operation conditions and the number of photons in the cavity mode provide the unique opportunity to study nonlinear effects in a quantum system. Here we explore such effects by coupling a fraction of the emitted light back into the cavity mode of feedback-coupled quantum-dot microcavity lasers with output powers in the sub-μW range. Using correlation spectroscopy, we demonstrate that feedback-coupling of emission via an external mirror can substantially affect the performance—and the photon statistics—of such microlasers. Interestingly, this type of self-feedback has been studied extensively for mW semiconductor lasers (SCL), where it can lead to a chaotic waveform. Chaotic lasers have been used to demonstrate high-bandwidth transmission of messages hidden in complex optical waveforms [11] , [12] , [13] and may lead to new forms of private and public channel cryptosystems [14] , [15] , [16] , as well as being a source for physical random number generators towards terahertz rates [17] , [18] , [19] , [20] . Thus, in our work, we merge two important fields of modern physics, namely nonlinear-optics of chaotic lasers and nanophotonics by studying the emission features of quantum-dot microlasers subject to an external feedback. Samples and experimental setup The system under study consists of electrically driven micropillar lasers with a single, low-density layer of In 0.3 Ga 0.7 As QDs as gain medium ( Fig. 1a , see Methods for details) [21] . The experiments were carried out at low temperature (20K) by means of high-resolution micro-electroluminescence (μEL) spectroscopy. The setup is equipped with a Michelson interferometer and a Hanbury-Brown and Twiss (HBT) configuration to measure the photon autocorrelation functions g (1) ( τ ) and g (2) ( τ ), respectively ( Fig. 1b ). The time resolution of the HBT is approximately 40 ps. The external cavity is formed of a mirror and a 90/10 beam-splitter, where the length is set to 3.48 m that corresponds to the round-trip time of the signal of τ ext =11.6 ns significantly larger than the coherence time of the lasers (see below). 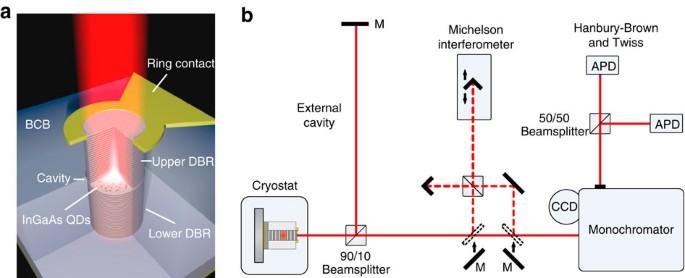Figure 1: Schematic of micropillar laser and experimental setup. (a) Schematic view of an electrically contacted micropillar laser structure. (b) Sketch of the experimental setup. The μEL signal can be analysed with a Michelson interferometer and a Hanbury-Brown and Twiss setup equipped with fibre-coupled Si-based avalanche photodiodes. Figure 1: Schematic of micropillar laser and experimental setup. ( a ) Schematic view of an electrically contacted micropillar laser structure. ( b ) Sketch of the experimental setup. The μEL signal can be analysed with a Michelson interferometer and a Hanbury-Brown and Twiss setup equipped with fibre-coupled Si-based avalanche photodiodes. Full size image Emission spectra of the microlaser The fundamental emission mode HE 11 of a micropillar with a perfect circular cross-section is double degenerate. This degeneracy is lifted for an elliptically shaped cross-section, and two orthogonal, linearly polarized emission modes appear [22] . 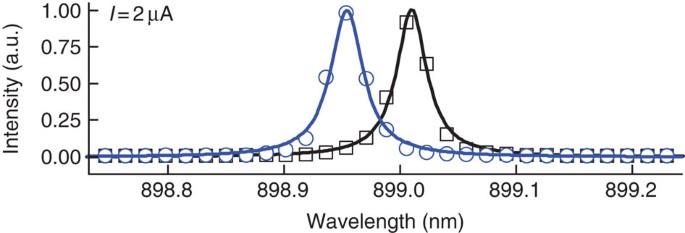Figure 2: Emission spectra of a micropillar laser. Polarization resolved μEL emission spectra of a micropillar laser with a diameter of 3.6 μm for an injection current of 2 μA (without feedback coupling). Due to a slight asymmetry of the micropillar cross-section, the fundamental cavity mode is split into two orthogonal linearly polarized components (mode A, black trace, at 0° and mode B, blue trace, at 90°, detection angle). Figure 2 shows polarization-resolved emission spectra of a micropillar laser with diameter of 3.6 μm at an injection current of 2 μA. Due to a slight asymmetry of the cross-section, two linearly polarized emission modes A (0° detection angle) and mode B (90° detection angle) can be resolved. The splitting between the two mode components amounts to about 0.07 nm. Figure 2: Emission spectra of a micropillar laser. Polarization resolved μEL emission spectra of a micropillar laser with a diameter of 3.6 μm for an injection current of 2 μA (without feedback coupling). Due to a slight asymmetry of the micropillar cross-section, the fundamental cavity mode is split into two orthogonal linearly polarized components (mode A, black trace, at 0° and mode B, blue trace, at 90°, detection angle). 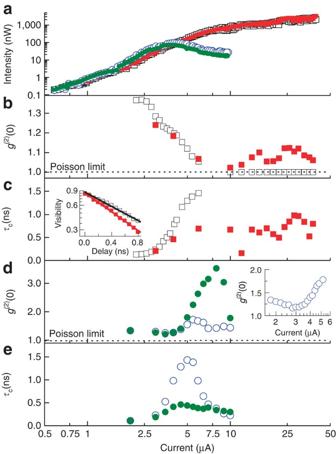Figure 3: Input-output characteristics and second-order photon autocorrelation functions. (a) Input-output characteristics of two linearly polarized HE11mode components (open square: mode A w/o fb, red square: mode A with fb, open circle: mode B w/o fb, green circle: mode B with fb) of a 3.6 μm diameter micropillar. (b) Second-order photon autocorrelation functiong(2)(0) for mode A with (red square) and without (open square) optical feedback versus injection current. (c) Width of the bunching signal for mode A (open square: w/o fb, red square: with fb). Inset: Visibility curvesV(τ) obtained from interferometric measurements on a 3.6 μm diameter micropillar above threshold. External feedback affects the coherence properties of the microlaser and leads to a decrease of the coherence time from 1.00 to 0.76 ns. (d) Second-order photon autocorrelation functiong(2)(0) for mode B with (green circle) and without (open circle) optical feedback versus injection current. The inset shows an additional, more detailed measurement ofg(2)(0) without feedback. (e) Width of the bunching signal for mode B (open circle: w/o fb, green circle: with fb). Full size image Input-output characteristics Figure 3a presents the input-output characteristics of the two linearly polarized fundamental HE 11 cavity mode components, mode A and mode B, of the micropillar laser with a diameter of 3.6 μm ( Fig. 2 ). The cavity mode is energetically split into two orthogonal components, owing to a slight elliptical asymmetry of the pillar. Mode A shows a smooth s-shaped dependence of the output power as a function of the injection current I inj , which is a clear indication of high-β lasing [23] . Mode B also enters the lasing regime, which can be seen by the nonlinear increase in the output power at I inj =2 μA. In this case, the output intensity saturates for I inj ≈4 μA and even drops with increasing injection current. The latter can be attributed to a gain competition between both modes, given that only about 10 QDs contribute effectively to the lasing action in these microlasers [10] . Note that applying an incoherent optical feedback to the micropillar has practically no effect on the average output intensity of either the mode or the threshold currents. This is consistent with SCLs, where feedback changes the temporal waveform, but not the average output intensity [24] . Figure 3: Input-output characteristics and second-order photon autocorrelation functions. ( a ) Input-output characteristics of two linearly polarized HE 11 mode components (open square: mode A w/o fb, red square: mode A with fb, open circle: mode B w/o fb, green circle: mode B with fb) of a 3.6 μm diameter micropillar. ( b ) Second-order photon autocorrelation function g (2) (0) for mode A with (red square) and without (open square) optical feedback versus injection current. ( c ) Width of the bunching signal for mode A (open square: w/o fb, red square: with fb). Inset: Visibility curves V ( τ ) obtained from interferometric measurements on a 3.6 μm diameter micropillar above threshold. External feedback affects the coherence properties of the microlaser and leads to a decrease of the coherence time from 1.00 to 0.76 ns. ( d ) Second-order photon autocorrelation function g (2) (0) for mode B with (green circle) and without (open circle) optical feedback versus injection current. The inset shows an additional, more detailed measurement of g (2) (0) without feedback. ( e ) Width of the bunching signal for mode B (open circle: w/o fb, green circle: with fb). Full size image Photon autocorrelation measurements of mode A The effect of optical feedback was further investigated by second order photon autocorrelation measurements over the whole current range. 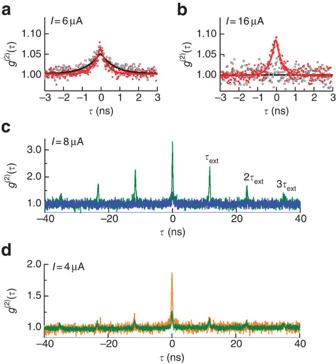Figure 4: Second-order photon autocorrelation functions under different operation conditions. (a) Correlation traces for mode A (open square: w/o fb, red square: with fb) for a current of 6 μA, where the width of the bunching signal is decreased by optical feedback. (b) Correlation traces for mode A (open square: w/o fb, red square: with fb) for a current of 16 μA, where bunching occurs only due to feedback. (c) Correlation traces for mode B with feedback (green curve) and without feedback (blue curve) for a current of 8 μA, depicting strong bunching and revival peaks with the round trip timeτextin the external cavity for optical feedback. (d) Correlation traces for mode B for a current of 4 μA with complete feedback (green curve) and with feedback from mode A only (orange curve) where theg(2)(0) value is enhanced due to the higher instability of mode B. An exemplary dataset of g (2) ( τ ) with and without feedback for I inj =6 μA is presented in Figure 4a . The photon correlation traces were fitted by a convolution of an idealized expression for bunching g (2) ( τ )=1+ b exp(− 2τ/τ c ) ( b : bunching amplitude, τ c : coherence time) and a Gaussian function of width 2 σ =40 ps, taking into account the time resolution of the HBT setup [5] . The deconvoluted g (2) (0) values for mode A with and without feedback are plotted in Figure 3b versus the injection current. For both cases, a clear transition from thermal to coherent emission was observed, as evidenced by a decrease of the g (2) (0) values from 1.36 to the Poisson limit of 1 above threshold [5] . The onset of lasing is also reflected in the strong increase of the coherence time from 0.13 to 1.47 ns ( Fig. 3c ). At the transition from spontaneous to stimulated emission, that is, in the current range between 2.0 and 7.5 μA, feedback does not affect the output intensity and g (2) (0) values ( Fig. 3a,b ). By contrast, the corresponding coherence times extracted from the photon autocorrelation measurements do depend on the feedback, as can be seen in Figure 3c . Here the width of the bunching signal is significantly decreased in the presence of self-feedback. This observation is consistent with measurements of the coherence time τ c that represents an important parameter of microlasers. Close to threshold, τ c increases strongly from values on the order of 10 ps to values exceeding 1 ns owing to the transition from predominantly spontaneous emission to stimulated emission [5] , [25] . Coherence times of another electrically pumped micropillar laser with a diameter of 3.6 μm were determined by a Michelson interferometer. The visibility V ( τ )=( I max − I min )/( I max + I min )=| g (1) ( τ )| with the maximum and minimum intensity of the interference fringes and the first-order field correlation function g (1) ( τ )=〈 E *( t ) E ( t + τ )〉/〈 E 2 ( t )〉 allow one to determine τ c via V ( τ ) α exp [ −|τ|/τ c ] [25] . Figure 3c (inset) shows visibility curves V ( τ ) of the microlaser above threshold with and without feedback. It is clearly seen that self-feedback disturbs laser action and leads to a decrease of the coherence time from 1.00 to 0.76 ns. Figure 4: Second-order photon autocorrelation functions under different operation conditions. ( a ) Correlation traces for mode A (open square: w/o fb, red square: with fb) for a current of 6 μA, where the width of the bunching signal is decreased by optical feedback. ( b ) Correlation traces for mode A (open square: w/o fb, red square: with fb) for a current of 16 μA, where bunching occurs only due to feedback. ( c ) Correlation traces for mode B with feedback (green curve) and without feedback (blue curve) for a current of 8 μA, depicting strong bunching and revival peaks with the round trip time τ ext in the external cavity for optical feedback. ( d ) Correlation traces for mode B for a current of 4 μA with complete feedback (green curve) and with feedback from mode A only (orange curve) where the g (2) (0) value is enhanced due to the higher instability of mode B. Full size image So far we have discussed the effect of self-feedback on the emission properties of the microlasers that are close to threshold. In this regime, when spontaneous emission of the gain medium dominates, the back-coupled signal is not strong enough to noticeably modify the photon statistics. The situation changes for injection currents exceeding the threshold value—an effect which is illustrated in Figures 3b and 4b . Indeed, in the region where thermal bunching disappears, namely for I inj >10 μA, a qualitative change in photon bunching is clearly seen with self-feedback. An illustrative correlation trace is depicted in Figure 4b for a current of 16 μA. Note that bunching associated with self-feedback ( g (2) (0)-values between 1.02 and 1.12) is observable up to about 18 times the lasing threshold current and should be distinguished from thermal bunching. In fact, it is related to the formation of random output pulses when the laser action is disturbed by photons reflected back into the active layer—an effect that is discussed in more detail below. The width of this bunching signal is displayed in Figure 3c versus I inj and amounts to about 700 ps for I inj >6 μA. Photon autocorrelation measurements of mode B We next examine the characteristics of mode component B in detail. The second-order autocorrelation function g (2) (0) and the width of the bunching signal are shown in Figure 3d,e , respectively, as a function of the injection current. The inset in Figure 3d illustrates an additional more detailed measurement of the g (2) (0) function without feedback. Without feedback, mode B exhibits a similar transition from thermal bunching to the Poisson limit for currents between 2.0 and 3.5 μA when compared with mode A. Furthermore, the coherence time extracted from the g (2) ( τ ) data increases up to about 5 μA, when the output intensity of mode B saturates as a result of gain competition with the stronger mode A ( Fig. 3a ). For I inj >5 μA, the optical gain of the QDs is transferred into mode A that shows lasing action. Consequently, the intensity of mode B decreases, and g (2) (0) increases up to values close to the thermal limit of 2, indicating a transition back to thermal emission. This interpretation is also supported by the coherence time, which drops for currents exceeding 5 μA. A striking feature is observed when feedback is applied to mode B in this transition regime: in the presence of self-feedback, photon bunching is drastically enhanced and values as high as g (2) (0)=3.51±0.06 are measured for a current of 8 μA, where the corresponding g (2) ( τ ) curves with and without self-feedback are presented in Figure 4c . Photon bunching with g (2) (0)>2 has been predicted to be a signature of superradiance of QDs and the associated emission of random light pulses [26] . However, in our system the observed super-thermal bunching depends on specific feedback and pump current conditions and therefore cannot be explained by a superradiance of QDs. Rather than this, the super-thermal bunching is associated with the subtle interplay between the two emission modes and random fluctuations in the output intensity of the feedback-coupled high-β microlaser. In fact, the maximal g (2) (0)-value for mode B is observed when the ratio of the intensities of mode A and mode B is roughly 10 2 , that is, most of the photons emitted from the QDs are funnelled into mode A. Note that for this type of micropillar, the number of QDs participating in the lasing action is typically on the order of ten [10] . The external feedback disturbs the lasing action of mode A, and the two modes now compete for the limited gain provided by the low number of QDs that initiates large and presumably chaotic intensity fluctuations in the output intensity of the two modes. Nevertheless, the relative fluctuations in mode B are expected to be larger than for mode A, as a fewer number of photons are coupled into this mode. This clearly explains why the measured g (2) (0)-values are much higher for the weaker mode B than for the stronger mode A. The decrease of the g (2) (0)-values between 8–10 μA ( cf . Fig. 3d ) can be attributed to a disturbance of the photon statistics of mode B by emission from mode A. With an increasing ratio between the intensities of mode A and B for I inj >5 μA, mode A (with g (2) (0) < ∼ 1.1) cannot be fully suppressed anymore when measuring the photon statistics of mode B. This affects the photon statistics of the detected signal and explains the decrease of g (2) (0) observed in Figure 3d for I inj > ∼ 8 μA. Furthermore, there are also revival peaks of the bunching symmetric to the peak at τ =0 in integer multiplications of the round trip time of the external cavity ( Fig. 4c,d ), which is a typical feature of chaotic SCL with self-feedback [27] . Simultaneously, Figure 3a indicates that the output intensity with and without feedback is almost the same. The fact that the time-averaged output intensity is independent of the feedback, along with the occurrence of pronounced bunching for mode B, is a strong indication that the temporal waveform of mode B consists of random spikes. This is strikingly similar to chaotic SCL, where a spiking waveform on a timescale of 100 ps evolves due to feedback [27] . Additional calculations of the autocorrelation function g (2) ( τ )=〈 I ( t ) I ( t + τ )〉/〈 I ( t )〉 2 from simulated spiking patterns [28] following the Lang-Kobayashi equations lead to pronounced bunching at τ =0. Solving these equations numerically, we obtain the emission intensity I ( t ) with the pump current I / I th , the external roundtrip time τ ext and the feedback rate κ acting as parameters. 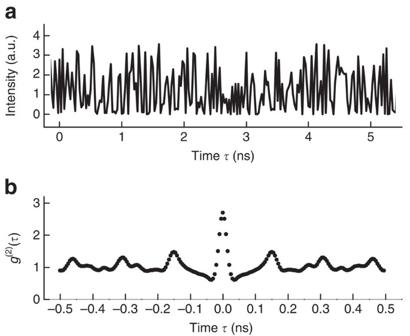Figure 5: Emission features and second-order autocorrelation function of a semiconductor laser. (a) Calculated emission intensityI(t) and (b) associated second-order autocorrelation functiong(2)(τ) of a semiconductor laser with self-feedback. Figure 5a shows the calculated emission intensity for I / I th =1.5, τ ext =10 ns and κ =10 ns −1 . As a result of self-feedback, the model predicts chaotic intensity fluctuations—a feature which has been observed experimentally for SCLs [19] , [27] , [29] . The related g (2) ( τ ) function is depicted in Figure 5b . The chaotic intensity fluctuations and the spiked emission of photons result in pronounced bunching with g (2) (0)>2. Thus, these calculations strongly support our interpretation of the experimental g (2) (0)-values in Figures 3 and 4 in terms of a spiked emission of the feedback-coupled micropillar lasers. Interestingly, the width of this bunching signal corresponds roughly to the average spike widths. On the basis of our measured bunching widths, this suggests that the spiking in our system also occurs on a time scale of a few hundred picoseconds. Figure 5: Emission features and second-order autocorrelation function of a semiconductor laser. ( a ) Calculated emission intensity I ( t ) and ( b ) associated second-order autocorrelation function g (2) ( τ ) of a semiconductor laser with self-feedback. Full size image Interaction of modes Our results indicate an interaction between both modes in the dynamics of the cavity, where they compete for the limited available resources provided by the QD gain medium. To confirm this picture, we performed a further experiment under linearly polarized feedback. Figure 4d shows correlation traces measured for mode B for I inj =4 μA for unpolarized and polarized feedback in the direction of mode A, respectively. Both cases exhibit bunching in mode B where an enhancement of photon bunching is observed when feedback is coupled selectively to mode A ( Fig. 4d , orange trace). This enhancement is attributed to short time fluctuations in mode A that induce large intensity fluctuations in mode B, as the total intensity does not change significantly. The weak mode mainly amplifies fluctuations of mode A which explains the higher g (2) (0) value under polarized feedback. The emergence of chaotic fluctuations in mW SCLs with time-delayed feedback is well described by deterministic rate equations, the Lang-Kobayashi equations [30] . However, for sub μW lasers, there are two additional sources of fluctuations preventing a possible mathematical description by rate equations. The first one is related to a typical intensity fluctuation expected to occur on a sub-nanosecond time scale, with at most O(10 2 ) photons, inducing fluctuations in the fraction of photons reflected back and re-entering the microlaser. The second source is the low number of QDs ( ∼ 10) being effectively involved in the lasing operation [10] . The robustness of the chaotic lasing phenomenon, with respect to quantum noise where a description by rate equations [30] is inconsistent, is of great interest from the point of view of nonlinear dynamics [31] , [32] . Our results give first insight into the chaotic behaviour of microlasers with self-feedback and have high potential to stimulate further experimental and theoretical studies. For instance, it will be important to find the correct description for the dynamics of micropillars with incoherent light feeding back into the cavity that will provide a better understanding of these super-thermal bunching phenomena. In this sense, our finding will bridge between two important fields of modern physics, namely nonlinear-optics and nanophotonics, which can pave the way for nanoscale physical random number generators and elements in advanced secure communication networks with synchronized chaotic intensities. Fabrication of the micropillar lasers The sample was grown by molecular beam epitaxy and is based on a one-λ thick GaAs cavity embedded in a lower n-doped distributed Bragg reflector with 27 GaAs/AlAs mirror pairs and an upper p-doped distributed Bragg reflector with 23 GaAs/AlAs mirror pairs. The gain was provided by a single layer of In 0.3 Ga 0.7 As QDs with a surface density of approximately 5×10 9 cm −2 . The micropillars were defined from the planar cavity in a subsequent electron beam lithography and dry chemical etching process. Then, the sample was planarized with the polymer benzocyclobutene and the upper Au ring contact was realized by a second electron beam lithography step. A detailed description of the fabrication process can be found in ref. 21 . How to cite this article: Albert, F. et al . Observing chaos for quantum-dot microlasers with external feedback. Nat. Commun. 2:366 doi: 10.1038/ncomms1370 (2011).